Galanin modulates the neural niche to favour perineural invasion in head and neck cancer Perineural invasion (PNI) is an indicator of poor survival in multiple cancers. Unfortunately, there is no targeted treatment for PNI since the molecular mechanisms are largely unknown. PNI is an active process, suggesting that cancer cells communicate with nerves. However, nerve–tumour crosstalk is understudied due to the lack of in vivo models to investigate the mechanisms. Here we developed an in vivo model of PNI to characterize this interaction. We show that the neuropeptide galanin (GAL) initiates nerve–tumour crosstalk via activation of its G protein-coupled receptor, GALR2. Our data reveal a novel mechanism by which GAL from nerves stimulates GALR2 on cancer cells to induce NFATC2-mediated transcription of cyclooxygenase-2 and GAL. Prostaglandin E2 promotes cancer invasion, and in a feedback mechanism, GAL released by cancer induces neuritogenesis, facilitating PNI. This study describes a novel in vivo model for PNI and reveals the dynamic interaction between nerve and cancer. Perineural invasion (PNI) predicts poor survival in head and neck squamous cell carcinoma (HNSCC), pancreatic, stomach and colon cancers [1] . PNI is associated with pain and tumour spread, independent of lymph or vascular involvement [2] . In contrast to previous assumptions, PNI is not a passive process that occurs via the path of least resistance or via the lymphatics [1] . Rather, the structure of the nerve and the occurrence of cancer within the nerve [1] , [3] suggest that PNI is an active process that requires invading cancer cells to degrade several layers of perineural sheath. PNI is observed in up to 80% of HNSCC cases and correlates with tumour recurrence and spread [4] , [5] . HNSCC can spread along the nerves into the brain or into sensory or motor nerves, and is associated with the loss of function, pain, numbness and formication, that is, the feeling of insects crawling under the skin [5] . HNSCC with PNI is treated aggressively but the prognosis remains poor. Unfortunately, there is no targeted treatment for PNI since the molecular mechanisms are largely unknown. Therefore, dissecting the mechanism of PNI is a critical area of research that would facilitate the development of novel therapeutics targeting PNI. Specific treatment of PNI would enhance patient survival and quality of life. Some oral cavity tumours exhibit a tendency towards neural invasion, whereas other tumours in similar locations do not invade nerves [2] . Therefore, it is likely that PNI requires specific biological interactions between HNSCC cells and nerves. In adenoid cystic carcinoma, a head and neck tumour that frequently exhibits PNI, neural invasion is correlated with the dysregulation of genes that regulate the release of neurotropic factors and adhesion molecules [6] . Although the altered neural microenvironment adjacent to tumours contributes to cancer progression, the limitations of existing in vivo models of PNI have hindered the understanding of nerve–tumour interactions [1] . To overcome this obstacle, we developed an in vivo model of PNI to characterize mechanisms of nerve–tumour interactions. We show that the neuropeptide galanin (GAL) initiates nerve–tumour crosstalk via activation of the G protein-coupled receptor galanin receptor 2 (GALR2) on cancer cells. GALR2 is also designated Galanin2 receptor or GAL 2 R ( www.guidetopharmacology.org ). Our data reveal that activated GALR2 induces nuclear factor of activated T cells, cytoplasmic, calcineurin-dependent-2 (NFATC2)-mediated transcription of cyclooxygenase-2 (COX2) and GAL. COX2 enzymatically facilitates prostaglandin E2 (PGE 2 ) production, promoting tumour progression. In a feedback mechanism, GAL released by cancer induces neuritogenesis and facilitates PNI. These studies demonstrate that the nerve initiates PNI via GAL, providing a potential treatment target. The novel approaches presented here further provide a starting point to investigate the roles of other neurotrophic proteins in PNI. 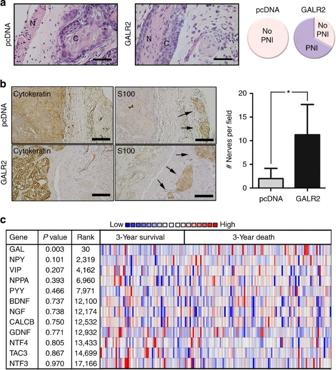Figure 1: GAL correlates with poor survival and neuronal involvement. (a) Murine tumours derived from OSCC3-GALR2 cells, but not control (OSCC3-pcDNA) cells, exhibit PNI (n=3 per group; scale bar, 100 μm; N=nerve; C=cancer). The complete image is inSupplementary Fig. 1b. Comparison of PNI with no PNI in control and GALR2-overexpressing murine xenografts (right panel). (b) GALR2-expressing murine tumours had more adjacent nerves than control tumours (n=3 per group, arrows identify nerves; scale bar, 50 μm). (*P<0.05, two-samplet-test; data represent mean+s.d.). Cytokeratin labels tumour and S100 labels nerves. GAL staining distal and proximal to the nerve is shown. (c) The Cancer Genome Atlas study shows that, of several neuronal proteins, only GAL DNA copy number significantly correlates with poor survival (two-samplet-test,P=0.003, 30th most significant). GALR2 promotes tumour progression Meta-analyses were conducted to compare the expression of neurotrophins and neuropeptides in HNSCC and normal (non-cancerous) samples ( Table 1 ). GAL (* P <0.02, one-sample t -test) and brain-derived neurotrophic factor (* P <0.025, one-sample t -test) were significantly overexpressed in HNSCC, whereas nerve growth factor, glial cell line-derived neurotrophic factor, neurotrophin-3, neuropeptide Y, peptide YY and vasoactive intestinal peptide were not upregulated. Details about the HNSCC studies, including accession number, weblink, reference and normal tissue used, are provided in Supplementary Table 1 . 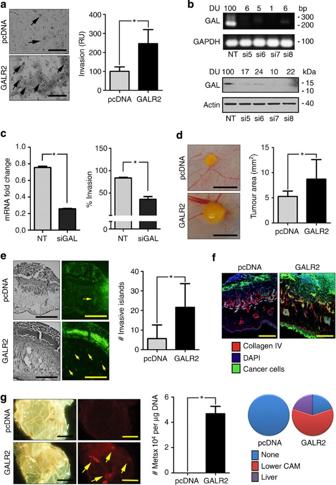Figure 2: GALR2 promotes tumour invasion and metastasis. (a) UM-SCC-1-GALR2 cells are more invasive than control UM-SCC-1-pcDNA cells in a Boyden chamber chemoinvasion assay with GAL as the chemoattractant (scale bar, 100 μm). Invasive cells (arrows) from both groups were quantified. Data are representative of three independent experiments with three replicates in each experiment. (*P<0.05, two-samplet-test; data represent mean+s.d.). (b) UM-SCC-1 cells were transfected with non-target (NT) siRNA or siGAL (#5, #6, #7, #8). Downregulation of GAL was verified in RNA (upper panel) and whole-cell lysates (lower panel) from these cells. (c) After verification of downregulation of GAL by qRT–PCR (left panel), CM from UM-SCC-1 (parent) cells transfected with NT siRNA or siGAL7 (siGAL) was used as the chemoattractant in a chemoinvasion assay performed with UM-SCC-1-GALR2 (right panel). Cells are significantly more invasive when stimulated with CM from UM-SCC-1-NT than from UM-SCC-1-siGAL7 cells. Data are representative of two experiments each with three replicates. (d–f) UM-SCC-1-GALR2 CAM tumours were (d) larger (scale bar, 5 mm), (e) more invasive (cancer cells are labelled green and highlighted by arrows, scale bar, 200 μm) and (f) more disruptive of the basement membrane than control (UM-SCC-1-pcDNA) tumours. Collagen IV and dashed lines label basement membrane (scale bar, 100 μm). (g) Metastases (yellow, arrows) from the upper CAM to the lower CAM were observed (scale bar, 5 mm). Metastases to the lower CAM and liver were also quantified with quantitative ALU-PCR. (pcDNA group: lower CAMn=4; livern=5; GALR2 group: lower CAMn=6, livern=6). The specific results for GAL, including the significance level in the individual studies and the meta-analysis, are included in Supplementary Table 2 . In 43 analyses of clinical samples from multiple cancers, high GAL expression was significantly correlated with poor clinical outcome ( Supplementary Fig. 1a ). 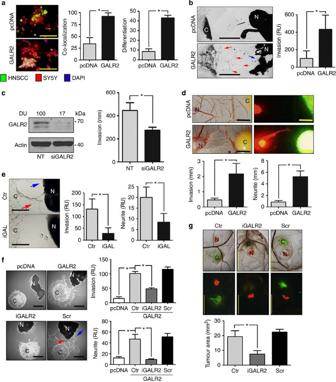Figure 3: GALR2 promotes PNI. (a) UM-SCC-1 cells (green) overexpressing GALR2 co-mingle with SH-SY5Y neuroblastoma cells (red) and induce more neuritogenesis (differentiation) than controls pcDNA, (two experiments, two replicates in each; scale bar, 100 μm). (b) UM-SCC-1-GALR2 cells are more invasive (red arrows) towards DRG than controls (UM-SCC-1-pcDNA) and induce neurite outgrowth (blue arrow; scale bar, 1 mm). (c) Knockdown of endogenous GALR2 in UM-SCC-1 cells, validated by immunoblot (left panel), inhibits invasion (right panel; two experiments, three replicates in each). (d) UM-SCC-1-GALR2 CAM tumours (green) are more invasive and induce neurite outgrowth (red; scale bar, 5 mm,n=6 in each group). (e) UM-SCC-1-GALR2 cell invasion (red arrow) and neurite outgrowth (blue arrow) are attenuated with antagonist anti-GAL antibody (iGAL; scale bar, 1 mm). (f) Invasion of UM-SCC-1-GALR2 (red arrow) and neurite outgrowth (blue arrow) are inhibited by M871 (designated iGALR2), but not scrambled peptide. (pcDNAn=3, GALR2n=6, GALR2-M871n=4, GALR2-Scrn=5; scale bar, 1 mm). (g) M871 (iGALR2) inhibits growth of UM-SCC-1-GALR2 CAM tumours (scale bar, 5 mm, Ctrn=7, iGALR2n=8, Scrn=8). Area was quantified with ImageJ.b,eare representative of three independent experiments with three replicates in each.fis representative of two experiments. (*P<0.05, two-samplet-test; graph represents mean+s.d.). The number of studies, cancer sites and number of clinical samples for each cancer is shown in Supplementary Table 3 . Table 1 Meta-analyses of neuropeptides. Full size table The neuropeptide GAL is the ligand for three G protein-coupled receptors—GALR1, GALR2 and GALR3. GALR2 is pro-proliferative [7] and is overexpressed in HNSCC due to a frequent chromosomal translocation [8] . Previously, we showed that GALR2 induces tumour growth in vivo [7] . Using sections from these murine tumours, we observed PNI in GALR2-overexpressing tumours but not in control tumours ( Fig. 1a , complete image in Supplementary Fig. 1b ). In addition, more nerves were present adjacent to GALR2-overexpressing murine tumours ( Fig. 1b , cytokeratin and S100 stains highlight cancer and nerves, respectively), suggesting that GALR2 induces neuritogenesis. Using DNA copy number, we found that high GAL predicted death at 3 years ( Fig. 1c ). Tachykinin-3, Neurotrophin-4 and Calcitonin-related polypeptide did not significantly differ in expression in any studies. Figure 1: GAL correlates with poor survival and neuronal involvement. ( a ) Murine tumours derived from OSCC3-GALR2 cells, but not control (OSCC3-pcDNA) cells, exhibit PNI ( n =3 per group; scale bar, 100 μm; N=nerve; C=cancer). The complete image is in Supplementary Fig. 1b . Comparison of PNI with no PNI in control and GALR2-overexpressing murine xenografts (right panel). ( b ) GALR2-expressing murine tumours had more adjacent nerves than control tumours ( n =3 per group, arrows identify nerves; scale bar, 50 μm). (* P <0.05, two-sample t -test; data represent mean+s.d.). Cytokeratin labels tumour and S100 labels nerves. GAL staining distal and proximal to the nerve is shown. ( c ) The Cancer Genome Atlas study shows that, of several neuronal proteins, only GAL DNA copy number significantly correlates with poor survival (two-sample t -test, P =0.003, 30th most significant). Full size image Invasion is essential for regional spread and metastasis. In HNSCC, GAL correlated with tumour-positive lymph nodes ( Supplementary Fig. 1c , upper panel) and tumour recurrence ( Supplementary Fig. 1c , lower panel), independent indicators of poor prognosis [9] . Therefore, we hypothesized that GAL may promote invasion via GALR2, an HNSCC phenotype that promotes tumour progression. To investigate this possibility in two independent HNSCC cell lines, we used the Boyden chamber chemoinvasion assay with GAL as the chemoattractant. Invasion was greater in cells overexpressing GALR2 than in control cells (pcDNA; Fig. 2a and Supplementary Fig. 2a ). Overexpression of GALR2 in UM-SCC-1 and OSCC3 cells was comparable to the physiologic levels of GALR2 in HNSCC cell lines ( Supplementary Fig. 2b,c ). To investigate whether GAL is required for the chemoinvasion observed in GALR2-expressing HNSCC cells, GAL was downregulated in parent UM-SCC-1 cells by siGAL and the conditioned medium (CM) from these cells was used for chemoinvasion assays with UM-SCC-1-GALR2 cells. Downregulation of GAL was verified by PCR and immunoblot ( Fig. 2b ). Short interfering RNA (siRNA)-mediated downregulation of GAL was also verified by quantitative reverse transcription–PCR (qRT–PCR; Fig. 2c , left panel). Downregulation of GAL lead to a significant reduction in invasion of HNSCC-GALR2 cells ( Fig. 2c , right panel). In contrast, growth medium with complete serum had no differential effect on control and GALR2-expressing HNSCC cells, consistent with GAL-specific effects. Figure 2: GALR2 promotes tumour invasion and metastasis. ( a ) UM-SCC-1-GALR2 cells are more invasive than control UM-SCC-1-pcDNA cells in a Boyden chamber chemoinvasion assay with GAL as the chemoattractant (scale bar, 100 μm). Invasive cells (arrows) from both groups were quantified. Data are representative of three independent experiments with three replicates in each experiment. (* P <0.05, two-sample t -test; data represent mean+s.d.). ( b ) UM-SCC-1 cells were transfected with non-target (NT) siRNA or siGAL (#5, #6, #7, #8). Downregulation of GAL was verified in RNA (upper panel) and whole-cell lysates (lower panel) from these cells. ( c ) After verification of downregulation of GAL by qRT–PCR (left panel), CM from UM-SCC-1 (parent) cells transfected with NT siRNA or siGAL7 (siGAL) was used as the chemoattractant in a chemoinvasion assay performed with UM-SCC-1-GALR2 (right panel). Cells are significantly more invasive when stimulated with CM from UM-SCC-1-NT than from UM-SCC-1-siGAL7 cells. Data are representative of two experiments each with three replicates. ( d – f ) UM-SCC-1-GALR2 CAM tumours were ( d ) larger (scale bar, 5 mm), ( e ) more invasive (cancer cells are labelled green and highlighted by arrows, scale bar, 200 μm) and ( f ) more disruptive of the basement membrane than control (UM-SCC-1-pcDNA) tumours. Collagen IV and dashed lines label basement membrane (scale bar, 100 μm). ( g ) Metastases (yellow, arrows) from the upper CAM to the lower CAM were observed (scale bar, 5 mm). Metastases to the lower CAM and liver were also quantified with quantitative ALU-PCR. (pcDNA group: lower CAM n =4; liver n =5; GALR2 group: lower CAM n =6, liver n =6). Full size image Using two cell lines in the chick embryo chorioallantoic membrane (CAM) model of HNSCC [10] , GALR2 promoted aggressive tumour growth and invasion in vivo . Tumours overexpressing GALR2 were larger ( Fig. 2d and Supplementary Fig. 2d ; n =6 per group, * P <0.05, two-sample t -test; data represent mean+s.d.) and more invasive ( Fig. 2e and Supplementary Fig. 2e ; n =6 per group, * P <0.05, two-sample t -test; data represent mean+s.d.) than controls, and destroyed the CAM basement membrane ( Fig. 2f and Supplementary Fig. 2f ). In addition, metastases to the lower CAM and liver of the embryos were increased in UM-SCC-1-GALR2 tumours compared with corresponding control tumours ( Fig. 2g ; pcDNA group: lower CAM n =4; liver n =5; GALR2 group: lower CAM n =6, liver n =6, * P <0.05, two-sample t -test; data represent mean+s.d.). GALR2 induces PNI Since the murine studies described above showed a correlation between GALR2 and PNI, we investigated the impact of GALR2 on PNI with additional models of neural–tumour interactions. Co-culture of UM-SCC-1 and SH-SY5Y human neuroblastoma cells led to neuritogenesis and co-mingling of the cells, which were significantly increased in GALR2-overexpressing cells ( Fig. 3a , * P <0.05, two-sample t -test; data represent mean+s.d.). Since SH-SY5Y is a neural tumour cell line, we also investigated GALR2-mediated interactions between HNSCC and normal (non-cancer) neural tissue using HNSCC cells co-cultured with rat dorsal root ganglia (DRG) explants. Both HNSCC-GALR2 cell lines tested were more invasive towards DRG and induced more neuritogenesis than control cells ( Fig. 3b and Supplementary Fig. 3a , * P <0.05, two-sample t -test; data represent mean+s.d.). Moreover, the downregulation of GALR2 with siRNA, as verified by immunoblot, inhibited cancer cell invasion towards DRG ( Fig. 3c , left and right panels, respectively, * P <0.05, two-sample t -test; data represent mean+s.d.). Figure 3: GALR2 promotes PNI. ( a ) UM-SCC-1 cells (green) overexpressing GALR2 co-mingle with SH-SY5Y neuroblastoma cells (red) and induce more neuritogenesis (differentiation) than controls pcDNA, (two experiments, two replicates in each; scale bar, 100 μm). ( b ) UM-SCC-1-GALR2 cells are more invasive (red arrows) towards DRG than controls (UM-SCC-1-pcDNA) and induce neurite outgrowth (blue arrow; scale bar, 1 mm). ( c ) Knockdown of endogenous GALR2 in UM-SCC-1 cells, validated by immunoblot (left panel), inhibits invasion (right panel; two experiments, three replicates in each). ( d ) UM-SCC-1-GALR2 CAM tumours (green) are more invasive and induce neurite outgrowth (red; scale bar, 5 mm, n =6 in each group). ( e ) UM-SCC-1-GALR2 cell invasion (red arrow) and neurite outgrowth (blue arrow) are attenuated with antagonist anti-GAL antibody (iGAL; scale bar, 1 mm). ( f ) Invasion of UM-SCC-1-GALR2 (red arrow) and neurite outgrowth (blue arrow) are inhibited by M871 (designated iGALR2), but not scrambled peptide. (pcDNA n =3, GALR2 n =6, GALR2-M871 n =4, GALR2-Scr n =5; scale bar, 1 mm). ( g ) M871 (iGALR2) inhibits growth of UM-SCC-1-GALR2 CAM tumours (scale bar, 5 mm, Ctr n =7, iGALR2 n =8, Scr n =8). Area was quantified with ImageJ. b , e are representative of three independent experiments with three replicates in each. f is representative of two experiments. (* P <0.05, two-sample t -test; graph represents mean+s.d.). Full size image The role of the nerve in tumour progression is relatively unknown due to the lack of appropriate in vivo models to characterize nerve–tumour interactions. To address this deficiency, we developed an in vivo model of PNI that demonstrates tumour neuritogenesis. In brief, a rat DRG was grafted onto the CAM and incorporated into the connective tissue. Subsequently, human HNSCC cells were introduced adjacent to the DRG. The grafted DRG is nourished by the developing vasculature of the CAM that replicates the pro-angiogeneic microenvironment observed in carcinogenesis. Tumour-nerve interactions are observed and quantified. Tumour cell invasion towards the nerve and neurite length were higher with HNSCC tumours overexpressing GALR2 than control tumours in both cell lines ( Fig. 3d and Supplementary Fig. 3b , * P <0.05, two-sample t -test; data represent mean+s.d.). To verify that GALR2 promotes neuritogenesis, we disrupted GAL-mediated GALR2 induction. When UM-SCC-1-GALR2 and DRG co-cultures were treated with anti-GAL antibody, cancer cell invasion and neuritogenesis were inhibited in vitro ( Fig. 3e ). Using a biochemical approach with M871, a peptide inhibitor against GALR2, similar inhibitory effects on invasion and neuritogenesis were observed ( Fig. 3f , * P <0.05, two-sample t -test; data represent mean+s.d.). A scrambled control peptide did not inhibit GALR2-mediated invasion or neuritogenesis ( Fig. 3f ). The inactivity of the control peptide was verified by its inability to inhibit ERK, a known target of GALR2 (ref. 7 ; Supplementary Fig. 3c ). In the CAM-DRG in vivo PNI model system, M871, but not the control peptide, inhibited tumour growth ( Fig. 3g ). These findings establish the importance of GAL-GALR2 in nerve–tumour interactions. GAL from nerve initiates nerve–tumour crosstalk GAL is secreted by both nerves and cancer cells [11] , [12] suggesting that nerve–tumour crosstalk may be initiated by the nerve or cancer. To rule out the possibility that autocrine stimulation of GALR2 by HNSCC-derived GAL alone drives PNI, we explored the role of neural-derived GAL in promoting invasion. To investigate this, CM from cultured rat DRG was incubated with anti-GAL antibody or IgG (control) to deplete GAL ( Fig. 4a , left panel). Depletion of GAL in the CM was verified by enzyme-linked immunosorbent assay (ELISA; Fig. 4a , right panel) before use in in vitro invasion assays. Invasion of UM-SCC-1-GALR2 cells was reduced when GAL was depleted compared with CM without depletion ( Fig. 4b , * P <0.05, two-sample t -test; data represent mean+s.d.). These findings show that neuronally derived GAL induces the invasion of HNSCC. 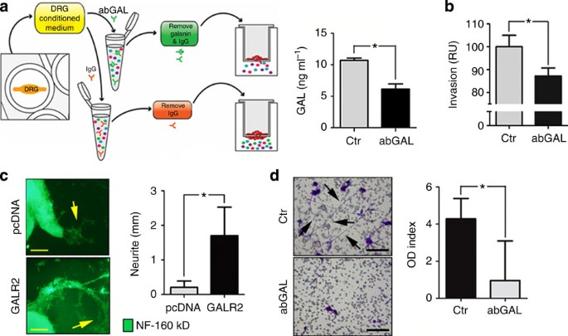Figure 4: GAL from both the DRG and tumour promote PNI. (a) Strategy to remove GAL from CM (left panel). Depletion is verified by ELISA (right panel). (b) CM was depleted of GAL by antibody and used as chemoattractant for UM-SCC-1-GALR2 cells in a modified Boyden chamber invasion assay, and less invasion is observed. (c) DRG treated with CM from UM-SCC-1-GALR2 cells have more neuritogenesis (arrows) than DRG treated with CM from UM-SCC-1-pcDNA cells (scale bar, 1 mm). Neurite extensions were quantified (right panel). (d) SH-SY5Y neuroblastoma cells extend more neurites (arrows) when treated with CM from UM-SCC-1-GALR2 cells than when GAL was depleted. (For all studiesn=3 per group; scale bar, 100 μm; *P<0.05, two-samplet-test, data represent mean+s.d.). Figure 4: GAL from both the DRG and tumour promote PNI. ( a ) Strategy to remove GAL from CM (left panel). Depletion is verified by ELISA (right panel). ( b ) CM was depleted of GAL by antibody and used as chemoattractant for UM-SCC-1-GALR2 cells in a modified Boyden chamber invasion assay, and less invasion is observed. ( c ) DRG treated with CM from UM-SCC-1-GALR2 cells have more neuritogenesis (arrows) than DRG treated with CM from UM-SCC-1-pcDNA cells (scale bar, 1 mm). Neurite extensions were quantified (right panel). ( d ) SH-SY5Y neuroblastoma cells extend more neurites (arrows) when treated with CM from UM-SCC-1-GALR2 cells than when GAL was depleted. (For all studies n =3 per group; scale bar, 100 μm; * P <0.05, two-sample t -test, data represent mean+s.d.). Full size image Since HNSCC also secrete GAL, we investigated whether, in a feedback loop, GAL released by HNSCC cells induce neurite formation. SH-SY5Y cells projected more neurites when incubated with CM from OSCC3-GALR2 cells compared with CM from control (OSCC3-pcDNA) cells ( Supplementary Fig. 3d ). In an investigation using DRG explants, CM from two tumour-GALR2 cell lines induced more neuritogenesis than control (pcDNA) CM ( Fig. 4c and Supplementary Fig. 3e , * P <0.05, two-sample t -test; data represent mean+s.d.). In addition, CM from UM-SCC-1-GALR2 cells was used as a chemoattractant to induce SH-SY5Y neuritogenesis through a porous membrane. When GAL was depleted in the CM from HNSCC cells using the strategy shown in Fig. 4a , fewer neurite projections were observed and quantified ( Fig. 4d left and right panels, respectively, * P <0.05, two-sample t -test; data represent mean+s.d.). Taken together, these findings support the hypothesis that GAL secreted from DRG and cancer induces invasion and neuritogenesis, respectively. GALR2 mediates invasion in HNSCC via NFATC2-induced COX2 Activation of GALR2 induces ERK and calcium signalling in cancer and neurons, leading to increased proliferation and survival [7] , [13] . Increased intracellular calcium and ERK activation lead to the induction and nuclear translocation of NFATC2, a transcription factor that induces transcription of pro-inflammatory cytokines [14] . Since GALR2 induces ERK [7] , we investigated GALR2’s role in NFATC2 activation. NFATC2 expression was higher in multiple HNSCC cell lines compared with primary human oral keratinocytes ( Fig. 5a , left upper panel). Moreover, GAL induced NFATC2 in HNSCC-GALR2 cells and to a much smaller extent in HNSCC-pcDNA control cells ( Fig. 5a , left lower panel). In two independent HNSCC-GALR2 cell lines, GAL induced the nuclear translocation of NFATC2 ( Fig. 5a right panel and Supplementary Fig. 4a ). Histone 2 (H2) and GAPDH were used as loading controls for nuclear and cytoplasmic proteins, respectively ( Fig. 5a , right panel). si8 was selected from a panel of four individual siRNAs due to its efficiency in downregulating NFATC2 ( Supplementary Fig. 4b ). In functional assays in UM-SCC-1-GALR2 and OSCC3-GALR2 cells, siNFATC2 reduced proliferation ( Fig. 5b and Supplementary Fig. 4c , * P <0.05, two-sample t -test; data represent mean+s.d.) and invasion ( Fig. 5c and Supplementary Fig. 4d , * P <0.05, two-sample t -test; data represent mean+s.d.). To verify that the functional impact of GALR2 is NFATC2 dependent, two clones of cells stably transduced with shNFATC2 were used. Stable downregulation of NFATC2 inhibited proliferation, whereas shNFATC2-1, which did not exhibit downregulation of NFATC2 ( Supplementary Fig. 4e ), proliferated at the same rate as cells transduced with the empty vector ( Supplementary Fig. 4f ). The in vitro findings of NFATC2 on proliferation were validated in vivo on the CAM. Downregulation of NFATC2 in UM-SCC-1-GALR2 cells decreased tumour growth ( Fig. 5d ) and invasion ( Fig. 5e ) compared with the same cells with scrambled short hairpin RNA (shRNA). Moreover, downregulation of NFATC2 prevented invasion of the basement membrane, which was not observed with scrambled shRNA ( Fig. 5f , * P <0.05, two-sample t -test; data represent mean+s.d.). NFATC2 knockdown disrupted the neural–tumour interactions in vitro and reduced HNSCC invasion towards the DRG ( Fig. 5g and Supplementary Fig. 4g , * P <0.05, two-sample t -test; data represent mean+s.d.). In contrast to UM-SCC-1-GALR2 cells, knockdown of NFATC2 in control UM-SCC-1-pcDNA (empty vector) cells did not have a significant impact on invasion towards the DRG ( Supplementary Fig. 4h , * P <0.05, two-sample t -test; data represent mean+s.d.). 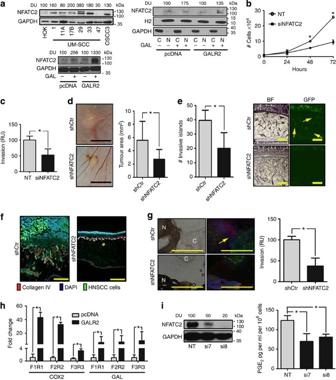Figure 5: GALR2 promotes tumour progression and PNI via NFATC2. (a, left upper panel) Multiple HNSCC cell lines express more NFATC2 than primary human oral keratinocytes (HOK); (a, left lower panel) UM-SCC-1-GALR2 and UM-SCC-1-pcDNA cells were induced with 5 nM GAL for 2 min and whole-cell lysates were immunoblotted with anti-NFATC2. GAPDH was used as a loading control; (a, right panel) GAL (5 nM) induces nuclear translocation of NFATC2 in UM-SCC-1-GALR2 and UM-SCC-1-pcDNA cells. H2 (histone 2), and GAPDH were used as loading controls for nuclear and cytoplasmic proteins, respectively. (b,c) UM-SCC-1-GALR2 cells transfected with siNFATC2, show reduced proliferation (b) and invasion (c) compared with the same cells transfected with NT siRNA. In CAM, UM-SCC-1-GALR2 cells with constitutive knockdown of NFATC2 (shNFATC2) induce tumours that are (d) smaller, (scale bar, 5 mm), (e) less invasive (arrows show invasive islands; scale bar, 200 μm; *P<0.02, two-samplet-test) and (f) less disruptive to the basement membrane (labelled with Collagen IV; scale bar, 200 μm) than the same cells with control scrambled shRNA (shCtr). (g) UM-SCC-1-GALR2-shNFATC2 cells exhibit less PNI than controls (cancer cells labelled ‘C’ fluoresce green and DRG are labelled ‘N’; arrow identifies neurite growth; scale bar, 1 mm). Graph shows quantification. (h) NFATC2 binds more to the promoter regions of PTGS2 (COX2) and GAL (GAL) in UM-SCC-1-GALR2 cells compared with control pcDNA. (i) When NFATC2 is downregulated with siRNA in UM-SCC-1-GALR2 cells, PGE2secretion decreases. For CAM experiments,n=6 for both;in vitroand DRG explant data are representative of three independent experiments each with three replicates. (*P<0.05, two-samplet-test; data represent mean+s.d.). Figure 5: GALR2 promotes tumour progression and PNI via NFATC2. ( a , left upper panel) Multiple HNSCC cell lines express more NFATC2 than primary human oral keratinocytes (HOK); ( a , left lower panel) UM-SCC-1-GALR2 and UM-SCC-1-pcDNA cells were induced with 5 nM GAL for 2 min and whole-cell lysates were immunoblotted with anti-NFATC2. GAPDH was used as a loading control; ( a , right panel) GAL (5 nM) induces nuclear translocation of NFATC2 in UM-SCC-1-GALR2 and UM-SCC-1-pcDNA cells. H2 (histone 2), and GAPDH were used as loading controls for nuclear and cytoplasmic proteins, respectively. ( b , c ) UM-SCC-1-GALR2 cells transfected with siNFATC2, show reduced proliferation ( b ) and invasion ( c ) compared with the same cells transfected with NT siRNA. In CAM, UM-SCC-1-GALR2 cells with constitutive knockdown of NFATC2 (shNFATC2) induce tumours that are ( d ) smaller, (scale bar, 5 mm), ( e ) less invasive (arrows show invasive islands; scale bar, 200 μm; * P <0.02, two-sample t -test) and ( f ) less disruptive to the basement membrane (labelled with Collagen IV; scale bar, 200 μm) than the same cells with control scrambled shRNA (shCtr). ( g ) UM-SCC-1-GALR2-shNFATC2 cells exhibit less PNI than controls (cancer cells labelled ‘C’ fluoresce green and DRG are labelled ‘N’; arrow identifies neurite growth; scale bar, 1 mm). Graph shows quantification. ( h ) NFATC2 binds more to the promoter regions of PTGS2 (COX2) and GAL (GAL) in UM-SCC-1-GALR2 cells compared with control pcDNA. ( i ) When NFATC2 is downregulated with siRNA in UM-SCC-1-GALR2 cells, PGE 2 secretion decreases. For CAM experiments, n =6 for both; in vitro and DRG explant data are representative of three independent experiments each with three replicates. (* P <0.05, two-sample t -test; data represent mean+s.d.). Full size image COX2 facilitates the formation of PGE 2 , a secreted protein important in tumour progression. Since NFATC2 induces pro-inflammatory mediators such as COX2 in lymphocytes and cancer [15] , the promoter regions of GAL (GAL) and PTGS2 (COX2) were interrogated and found to have NFATC2-binding sites. Using chromatin immunoprecipitation (ChIP), we validated that NFATC2 binds the promoter regions of PTGS2 and GAL ; binding was higher in UM-SCC-1-GALR2 cells than control cells ( Fig. 5h , * P <0.05, two-sample t -test; data represent mean+s.d.). Moreover, NFATC2 downregulation reduced COX2 expression ( Supplementary Fig. 4i ) and PGE 2 secretion in both HNSCC-GALR2 cell lines ( Fig. 5i and Supplementary Fig. 4j , * P <0.05, two-sample t -test; data represent mean+s.d.). Taken together, GALR2 induces PGE 2 secretion via NFATC2-mediated transcription of COX2. In a meta-analysis of multiple HNSCC studies, COX2 is upregulated in cancer compared with normal (non-cancer; Supplementary Fig. 5a in a one-sample t -test against the hypothetical mean of 0.05, P <0.0001). Details about the meta-analysis are given in Supplementary Table 4 . COX2 is highly expressed adjacent to nerves in most human HNSCC clinical tissue specimens with PNI ( Fig. 6a ; clinical data in Supplementary Table 5 ). In mice, 80% of HNSCC-GALR2 tumours expressed COX2 at the invasive front, whereas COX2 was not detected in control tumours ( Fig. 6b ). COX2 and endogenous GALR2 expression did not correlate in HNSCC cell lines ( Supplementary Fig. 5b ), likely because GALR2 expression may not reflect GALR2-induced signalling. More importantly, immunoblot and ELISA analyses demonstrate that HNSCC-GALR2 cells express more COX2 and secrete more PGE 2 than control pcDNA cells ( Fig. 6c and Supplementary Fig. 5c , * P <0.05, two-sample t -test; data represent mean+s.d.). HNSCC-GALR2 cells with siRNA-mediated COX2 knockdown ( Supplementary Fig. 5d , si6 and si8 selected) demonstrated reduced invasion compared with controls ( Fig. 6d and Supplementary Fig. 5e , * P <0.05, two-sample t -test; data represent mean+s.d.). 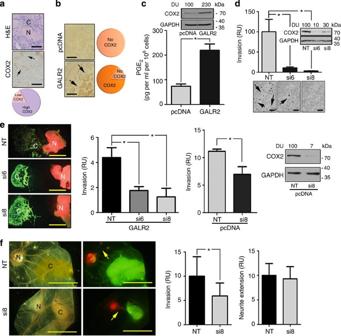Figure 6: COX2 regulates HNSCC progression but not neural–tumour crosstalk. (a) Most human tumours with PNI express high COX2 adjacent to nerves (arrows; scale bar, 100 μm). (N=nerve; C=cancer). (b) Most murine tumours with high GALR2 express COX2 at the invasive front (arrows; scale bar, 100 μm), but COX2 is not highly expressed by control tumours. (c) UM-SCC-1-GALR2 cells express more COX2 (immunoblot) and secrete more PGE2(ELISA) than control cells. (d) siCOX2 in UM-SCC-1-GALR2 cells decreases invasion (arrows label invasive cells; scale bar, 200 μm, immunoblot verifies knockdown). (e) Downregulation of COX2 decreases invasion of UM-SCC-1-GALR2 (immunofluorescence and left graph) and UM-SCC-1-pcDNA (right graph) cells towards DRG in co-culture. (scale bar, 1 mm; *P<0.02, two-samplet-test) (f) siRNA-mediated COX2 downregulation in UM-SCC-1-GALR2 tumours blocks cancer cell invasion (left graph), but does not affect the extension of DRG toward tumours (right graph; scale bar, 5 mm, arrows show neurites). For CAM experiments,n=6 per group andin vitroand DRG explant data are representative of three independent experiments each with three replicates. (*P<0.05, two-samplet-test; data represent mean+s.d.). (N=DRG; C=cancer). Figure 6: COX2 regulates HNSCC progression but not neural–tumour crosstalk. ( a ) Most human tumours with PNI express high COX2 adjacent to nerves (arrows; scale bar, 100 μm). (N=nerve; C=cancer). ( b ) Most murine tumours with high GALR2 express COX2 at the invasive front (arrows; scale bar, 100 μm), but COX2 is not highly expressed by control tumours. ( c ) UM-SCC-1-GALR2 cells express more COX2 (immunoblot) and secrete more PGE 2 (ELISA) than control cells. ( d ) siCOX2 in UM-SCC-1-GALR2 cells decreases invasion (arrows label invasive cells; scale bar, 200 μm, immunoblot verifies knockdown). ( e ) Downregulation of COX2 decreases invasion of UM-SCC-1-GALR2 (immunofluorescence and left graph) and UM-SCC-1-pcDNA (right graph) cells towards DRG in co-culture. (scale bar, 1 mm; * P <0.02, two-sample t -test) ( f ) siRNA-mediated COX2 downregulation in UM-SCC-1-GALR2 tumours blocks cancer cell invasion (left graph), but does not affect the extension of DRG toward tumours (right graph; scale bar, 5 mm, arrows show neurites). For CAM experiments, n =6 per group and in vitro and DRG explant data are representative of three independent experiments each with three replicates. (* P <0.05, two-sample t -test; data represent mean+s.d.). (N=DRG; C=cancer). Full size image COX2 downregulation disrupts PNI but not neuritogenesis COX2 is correlated with PNI in pancreatic cancer [16] . Given the importance of GALR2-mediated COX2 expression in invasion, the role of COX2 in mediating PNI was also investigated. The downregulation of COX2 reduced HNSCC cell invasion towards DRG in vitro in GALR2-overexpressing and control (pcDNA) cells ( Fig. 6e and Supplementary Fig. 5f , * P <0.05, two-sample t -test; data represent mean+s.d.). Importantly in vivo , siCOX2 inhibited the invasion of HNSCC towards DRG ( Fig. 6f , left graph, * P <0.05, two-sample t -test; data represent mean+s.d.) but did not significantly impact neurite growth towards the tumour ( Fig. 6f , right graph, * P <0.05, two-sample t -test; data represent mean+s.d.). Together these studies indicate that COX2 knockdown in HNSCC disrupts invasion towards neurons but does not inhibit tumour neuritogenesis. PNI is correlated with tumour recurrence, spread and poor survival in multiple cancers. Understanding PNI and targeting the regulatory mechanism is essential to improving survival. Using in vitro and a novel in vivo model, we focused on nerve–tumour interactions in HNSCC and showed that nerve-derived GAL initiates crosstalk between nerves and cancer cells by activating GALR2 in tumours. In turn, activated GALR2 induces NFATC2-mediated secretion of pro-inflammatory mediators and neuropeptides from tumour cells leading to invasion and neuritogenesis ( Fig. 7 ). GALR2-mediated PGE 2 secretion promotes invasion. Moreover, GAL secretion from the tumour cells induces neuritogenesis, thereby completing a feedback loop. Targeting GALR2 or GAL disrupted neural–tumour crosstalk, and blocked PNI and neuritogenesis. Thus, our findings establish that reciprocal communication between nerves and cancer cells occurs during PNI and suggest a target pathway to interrupt this crosstalk. 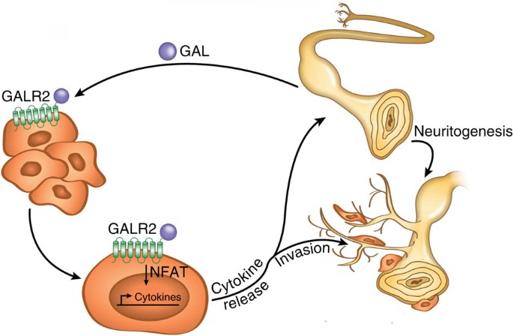Figure 7: A model of neural–tumour crosstalk mediated by the neuropeptide GAL. Neurons release GAL following injury or inflammation and activate tumour-expressed GALR2. GALR2 activation leads to NFATC2-mediated transcription and secretion of COX2/PGE2and GAL, thereby promoting PNI and neuritogenesis, respectively. Targeting GALR2 or GAL blocks PNI by disrupting neural–tumour crosstalk. Figure 7: A model of neural–tumour crosstalk mediated by the neuropeptide GAL. Neurons release GAL following injury or inflammation and activate tumour-expressed GALR2. GALR2 activation leads to NFATC2-mediated transcription and secretion of COX2/PGE 2 and GAL, thereby promoting PNI and neuritogenesis, respectively. Targeting GALR2 or GAL blocks PNI by disrupting neural–tumour crosstalk. Full size image The dynamic interaction between nerves and cancer cells is underexplored. It is likely that PNI requires specific biological interactions between HNSCC and nerves since HNSCC exhibits a tendency towards neural invasion, whereas some other head and neck cancers (for example, low-grade mucoepidermoid carcinoma) do not invade nerves [2] . Cancer cells establish connections with nerves (neural–neoplastic synapse), and are induced by neural factors [17] that impact metastasis [18] . Nerve–tumour interactions are implicated by clinical studies, for example, studies showing correlation between PNI and expression of nerve growth factor and its receptor, TrkA [19] , semaphorin 4D [20] and laminin-5 (ref. 21 ). Studies shown here support that GAL and GALR2 have a significant role in nerve–tumour interactions. GAL and GALR2 have actions in the neuronal system and in cancer, but possible roles in regulating crosstalk between nerves and cancer were previously not investigated. Human GAL is a 30-amino acid neuropeptide that regulates memory and has neurotrophic and neuroprotective roles [22] , [23] . Aside from well-characterized roles of GAL in nocioception and regeneration [24] , [25] , [26] , GAL is also implicated in non-neuronal contexts. For example, GAL is highly expressed in keratinocytes where it may have immune and proliferative functions [26] , and has abundant binding sites around dermal arteries, artiorioles and sweat glands where it may be involved in thermoregulation and the immune response [27] . GAL has an emerging mitogenic role in cancer [22] , for example, mice overexpressing GAL develop pituitary tumours [28] . GAL induces three G protein-coupled receptors—GALR1, GALR2 and GALR3. While GALR2 and GALR3 are pro-proliferative and promote survival [7] , [29] , GALR1 is a tumour suppressor [12] . In HNSCC, GAL is anti-proliferative via GALR1, and promotes aggressive tumour growth and survival via GALR2 (refs 7 , 12 ), that is, GALR1 and GALR2 have antagonistic effects. GALR1 is frequently deleted or silenced in HNSCC [30] , [31] , in effect enhancing GALR2-induced signalling. Thus, GALR2-induced signalling may be enhanced by the overexpression of GALR2 or by normal expression of GALR2 with concurrent downregulation of GALR1 (ref. 8 ). This may explain why endogenous GALR2 and COX2 expression are not correlated. Aside from roles in proliferation, cell survival and regeneration, GAL has a well-characterized role in nocioception [24] , [25] , [26] . Peripheral nerves release molecules that mediate pain and regeneration [32] , [33] . GAL is typically expressed at low levels in peripheral nerves but increases following injury and inflammation [34] , [35] . GAL mediates the regeneration and survival of inflamed nerves [36] . In fact, GAL and GALR2 (but not GALR1) are upregulated in lumbar and facial motor neurons after injury [37] , [38] . Consistent with these studies, we show that the GALR2-mediated release of GAL from HNSCC induces neuritogenesis. HNSCC is commonly associated with a prominent inflammatory response, which may induce nerves [39] , [40] . In a clinical context, the encroachment of nerves by an invading tumour, or transectioning the nerve while removing a tumour, or taking a surgical biopsy may stimulate GAL release by nerves, thereby initiating or enhancing nerve–tumour interactions. Thus, using a transected nerve on the CAM-PNI model simulates the clinical context by which an injured or inflamed nerve is primed to release neuropeptides, resulting in PNI and neuritogenesis. The significance of the primed neural niche in the tumour microenvironment has been alluded to through histopathological observation and three-dimensional reconstruction of tumours from labelled tissue sections [41] . However, the mechanisms of PNI are relatively unknown because previously developed in vitro models do not capture the impact of the dynamic involvement of the nerve in neural–tumour interactions [1] . Most in vivo studies of PNI focus on tumour spread and inhibition of motor function, and depend on direct tumour injection into sciatic nerves [42] . The sciatic nerve injection model is useful to demonstrate destructive tumour progression and pain resulting from tumour cells within nerves. However, in bypassing the invasive process and the proliferative or inductive roles of the nerve, these previous models do not truly replicate PNI. In a different approach, surgically implanted orthotopic tumour grafts were used to characterize the importance of β-adrenergic receptors in promoting PNI and prostate cancer progression [43] . The CAM-DRG in vivo model used in our study addresses the deficits of previous in vivo models by demonstrating neuronal outgrowth into the peritumoral niche. The system is also useful in studying therapy to disrupt PNI. The model can be used to evaluate response to treatment by measuring the response of the tumour and the nerve, both of which could promote tumour recurrence. PNI was disrupted chemically with the GALR2 antagonist M871 or with an antibody to GAL. The GAL-depletion method ( Fig. 4a ) allowed us to dissect the specific contributions of nerve-derived GAL to invasion and HNSCC-derived GAL to neoneuritogenesis, confirming that these processes involve reciprocal interaction and not autocrine activation of the nerve or tumour cells. This is important because both nerve and tumour cells secrete GAL [12] , [34] , [35] . These studies support the concept that therapies targeting GAL and GALR2 should be evaluated as the first potential anti-PNI therapies. Further investigations with this model will elucidate the role of various stromal tissues in promoting epithelial–mesenchymal transition, an important phenotype in many cancers [44] , [45] , [46] . An alternative model could have used xenografted tumours in GAL- or GALR2-knockout mice; however, developmental deficits in the neural tissue of these mice make this option unfavourable. The nerve is atrophic in GAL-knockout mice [47] . In GALR2-knockout mice, there is a 20% reduction in neurons in the DRG [48] , so changes observed in HNSCC may not represent alterations in GAL secretion or GALR2 signalling but rather an impact on the nerve itself. Since the knockdown of neuronal proteins such as GAL or GALR2 causes deficits in mice [47] , [49] , it was necessary to develop a model to evaluate the impact of these proteins on PNI using DRG from wild-type animals. NFATC2 is emerging as a key regulator of multiple cancer-promoting phenotypes [14] . GALR2 and NFATC2 have been independently shown to be important in cancer [50] , but their mechanism of action is poorly understood. In HNSCC, GALR2 activates ERK [7] and p38-MAPK to enhance angiogenesis and tumour growth [51] . In adrenal pheochromocytoma cells, GALR2 upregulates intracellular calcium [52] . These effectors stimulate calcineurin, which dephosphorylates (activates) NFATC2, thereby enabling NFATC2’s translocation to the nucleus. However, before this study, the role of GALR2 signalling in NFATC2-mediated PGE 2 secretion was not established. In Fig. 5a (upper panel), NFATC2 exhibits a variation in protein size and a doublet in some samples. This is likely due to variations in phosphorylation of NFATC2 since phosphorylation increases the molecular mass of this protein [53] . The doublet suggests that both phosphorylated and dephosphorylated NFATC2 are present. Since NFATC2 is a transcription factor, it is possible that its effects are independent of activation by GALR2. However, in contrast to GALR2 cells, knockdown of NFATC2 in control (empty vector) cells did not have a significant impact on invasion. Together these data support that the effect of NFATC2 knockdown is dependent on induction by GALR2. There is a spectrum of SCC with neural invasion, which ranges from those that are highly correlated with metastases to the lymph nodes [54] to those that spread to the brain stem but rarely to lymph nodes [55] . The spread of tumour cells into the brain and brain stem via the perineural space of the nerve is termed perineural spread [56] . There are well-documented studies showing the perineural spread of cutaneous SCC to the brain stem where the epi- and perineurium provided an excellent barrier to spread outside the nerve [56] . Perineural spread is not covered by our research, which focused on the spread of cancer towards and into the nerve. A diagnosis of PNI has long been informative to clinicians in treatment planning. A widely used definition of PNI is tumour that approximates the nerve, covering at least 33% of its circumference, or in one of the three layers of the nerve sheath [1] . These were the criteria used for analysis of mouse tissue sections in the current study. Another definition of PNI is perineural (within the perineural space), intraneural (invading endoneurium) and epineural (invading epineurium) tumour [56] . Given the layers of collagen and basement membrane that surround the nerve, and the increasing recognition that PNI is an active process [1] , it is likely that the cancer cells invade the epineurium, perineurium and endoneurium, to gain access to Schwann cells and axons. However, due to the variable course of nerves, it is challenging to determine conclusively on tissue sections the presence, extent of involvement and absolute number of nerves involved [56] . The CAM-nerve model, in which the nerves are visualized by fluorescence, is a valuable asset to the investigation of PNI. In human tissue, it is unclear how much the definition of PNI should be restricted or expanded to facilitate treatment planning. Features under consideration are depth of the nerves exhibiting PNI, presence of PNI beyond the invasive front of the tumour, and diameter of the nerves. Given the tumour-neural interaction shown here, additional considerations may be the distance of nerves from the tumour and neuritogenesis. Factors secreted by nerves bind to receptors on cancer cells to facilitate invasion into nerves. Precision medicine is a promising treatment-planning strategy that relies on molecular profiling to determine the optimal treatment strategy for each patient. Although PNI is linked to poor clinical outcome, there is no specific treatment for PNI. It is critical to identify the molecular fingerprint and understand the mechanism of neural–tumour interactions to identify novel PNI-specific treatment. Our study identifies the GALR2-induced pathway as a potential treatment target of PNI. Cell culture HNSCC cell lines UM-SCC-1 (from Thomas Carey, University of Michigan) and OSCC3 (from Peter Polverini, University of Michigan) were genotyped at the University of Michigan DNA Sequencing Core pre- and post completion of studies. Genotype was verified against published sequences for UM-SCC cell lines [57] and OSCC3 was compared with an early passage (P2) of cells. OSCC3 is thought to be derived from a squamous cell carcinoma of the ventral tongue [58] , [59] but HeLa cell contamination was recently identified [60] . Therefore, these cells may not be a pure HNSCC cell line. In this study, multiple cell lines and complementary approaches were used to elucidate the overall function of GALR2 in PNI. HNSCC cells and the neuroblastoma cell line SH-SY5Y (from Stephen K. Fisher, University of Michigan) were cultured in Dulbecco’s Modified Eagle Medium (DMEM, Gibco, 11965-092) supplemented with 10% fetal bovine serum (Gibco, 16000-044) and 1% PenStrep (Gibco, 15140-122). UM-SCC-1 and OSCC3 cells were transfected with pcDNA3.1 (Invitrogen, V790-20) and pcDNA3.1-GALR2 (Missouri S&T cDNA Resource Center, GALR200000). Geneticin (Gibco, 10131-027, 50 mg ml −1 ) was used to select and maintain stable colonies. UM-SCC-1 and OSCC3 cells transfected with pcDNA3.1-GALR2 were transfected with control non-targeting siRNA (Dharmacon, D-001810-10-05) or siRNA targeting NFATC2 (Dharmacon, LQ-003606-00) and COX2 (Dharmacon, LQ-004557-00-0002, siRNA sequences are listed in Supplementary Table 6 ). For stable NFATC2 knockdown, UM-SCC-1 and OSCC3 cells overexpressing GALR2 (UM-SCC-1-GALR2 and OSCC3-GALR2, respectively) were transduced with shRNA lentiviral particles (University of Michigan shRNA Core). Stable colonies were selected using Puromycin (Santa Cruz Biotechnology, sc-108071B, 10 μg ml −1 for UM-SCC-1 cells and 25 μg ml −1 for OSCC3 cells). Primary human oral keratinocytes isolated from oral mucosa (ScienCell Research Laboratories, 2610) were cultured according to the manufacturer’s instructions. Chromatin immunoprecipitation The EZ-Magna ChIP A/G kit (EMD Millipore, 17-10086) was used to perform ChIP as described [61] . An anti-NFATC2 antibody (Santa Cruz Biotechnology, sc-7296) and control rabbit IgG (Dako, X0936) were used. qRT–PCR was used to analyse purified DNA to determine relative fold enrichment compared to input DNA. The sequences of the Ptgs2 (COX2) and Gal (GAL) primers are provided in Supplementary Table 7 . Data analysis GraphPad Prism (GraphPad software) was used for statistics. A Student’s t -test was performed with a P value of <0.05 determined to be statistically significant. DRG organ culture Rat DRG and human HNSCC cells were co-cultured in Matrigel Basement Membrane Matrix (BD Biosciences, 356234), similar to a described method [3] . DRG were dissected from postnatal day-30 Sprague–Dawley rats within 1 h of euthanasia and placed in 15 μl of 4.6 mg ml −1 Matrigel. HNSCC cells (2 × 10 4 ) were seeded in an adjacent droplet of Matrigel, and cultures were immobilized by warming to 37 °C and cultured in DMEM (Gibco, 11965-092) supplemented with 10% fetal bovine serum (Gibco, 16000-044) and 1% PenStrep (Gibco, 15140-122). Cultures were maintained at 37 °C with 5% CO 2 for 2 days to observe cancer cell and neurite interactions. GALR2 inhibitor M871 (Tocris Biosciences, 2698), scrambled peptide (Thermo-Fisher Pierce Biotechnology, Rockford, IL) or dimethylsulphoxide control was used at 10 nM in culture or at 4 μM for CAM studies. Two scrambled peptides were generated (1: LALLYSGPELPLAPHAGNPATW; 2: TALGPLPLWPGLSYHAPNAAEL) and scrambled peptide 2 was used for CAM studies. GAL antibody and rabbit serum IgG were used at 3 ng ml −1 . Neurite extension and cancer cell movement were imaged after 48 h and quantified using ImageJ software (W.S. Rasband, NIH, Bethesda, MD; http://imagej.nih.gov/ij/ ). CM was prepared from rat DRG in DMEM (100 μl) without supplements; the supernatant was collected at 18 h, after centrifugation at 10,000 r.p.m. Efforts to reduce bias Protocols were developed to eliminate investigator bias in quantifying samples. Quantification was routinely performed by two individuals, one of whom was blinded to the hypothesized outcome. Whenever possible, objective quantification methods such as microplate readings and computer-based quantification of images were selected. ELISA for GAL CM from rat DRG (100 μl) was incubated with anti-GAL antibody (EMD Millipore, AB5909; 1:1000) or rabbit IgG (Dako, X0936) for 1 h at room temperature. For GAL-depletion studies, CM from human HNSCC cells was incubated with anti-GAL antibody (EMD Millipore, AB5909, 1:1000) or control rabbit IgG (Dako, X0936) for 1 h at room temperature. Conjugated GAL and unbound antibody or IgG were removed by centrifugation with an Amicon Ultra 50 K centrifugal filter (EMD Millipore, UFC805024) for 10 min at 4,000 r.p.m. GAL depletion was verified by ELISA (Peninsula Laboratories International, S-1208; detection range 0–10 ng ml −1 ) according to the manufacturer’s instructions using the standard curve provided. The CM was then used as a chemoattractant in the bottom chamber of the assay. PCR analysis of GAL transcript Cells transfected with siGAL were lysed with QIAzol and RNA was prepared with miRNeasy and RNase free DNase (Qiagen, 217004 and 79254). Complementary DNA (cDNA) was synthesized from 1 μg of RNA using SuperScript-II Reverse Transcriptase First-Strand Synthesis System (Invitrogen, 11904-018). cDNA was purified by Amicon filters (Millipore, UFC500324). To detect GAL expression, semi-quantitative PCR was performed with synthesized cDNA (50 ng) using primers: forward-5′-GCGCACAATCATTGAGTTTC′-3′; reverse-5′-GGCAAAGAGAACAGGAATGG-3′. PCR conditions were denaturation 95 °C for 5 min, annealing 55 °C for 5 min, 22 cycles of 95 °C for 30 s, 55 °C for 30 s, extension at 70 °C for 1 min and a final hold of 70 °C for 7 min. Platinum Taq (Invitrogen, 10966018) was used for all PCR reactions. As internal control, identical PCR reactions were performed using primers to GAPDH forward-5′-GCGAGATCCCTCCAAAATCAA-′3 and reverse-5′-GTTCACACCCATGACGAACAT′-3. PCR product was electrophoresed on a 1.5% agarose gel, stained with ethidium bromide (Sigma, E1510) and photographed. qRT–PCR qRT–PCR was performed with Power SYBR Green Master Mix (Applied Biosystems) using primers listed in Supplementary Table 7 . Data were analysed by the relative quantification method with normalization to GAPDH and then to normal keratinocytes [62] . ELISA for PGE 2 CM was collected from HNSCC cell lines UM-SCC-1 and OSCC3 at 60–70% confluence, in DMEM without any supplements; the supernatant was collected at 24 h, after centrifugation at 10,000 r.p.m. (ref. 12 ). The total number of cells was quantified with a Countess Cell Counter (Invitrogen, C10227). PGE 2 was quantified as a surrogate for COX2 using a competitive ELISA (R&D Systems, KGE004B) in three independent experiments per cell line. Human subjects After approval of exempt status by the University of Michigan Institutional Review Board, deidentified paraffin-embedded human HNSCC tissues were used for immunohistochemistry. Immunoblot Cells were lysed with 1% NP40 protein lysis buffer (50 mM Tris pH7.4, 1%NP40, 200 mM sodium chloride, 5 mM magnesium chloride, 10% glycerol). Protein (15–30 μg) was electrophoresed and transferred to a nitrocellulose membrane (0.1 μm, Fisher Scientific, 09-301-120), which was blocked in 5% non-fat dry milk in TBST (Tris-buffered saline with 0.01% Tween 20) except for the phosphoERK antibody, for which the nitrocellulose membrane was blocked in 5% bovine serum albumin in TBST. The following primary antibodies were incubated overnight at 4 °C: anti-GAL (EMD Millipore, AB5909; 1:500), anti-GALR2 (Alpha Diagnostics, GALR21-A; 1:250), anti-actin (BD Scientific, 612656; 1:1000), anti-NFATC2 (Sigma HPA008789, 1:500, Fig. 5a upper left panel and Supplementary Fig. 4a,b ; Cell Signalling Technologies 5861, 1:500, Fig. 5a right and lower left panels, Fig. 5i , Supplementary Fig. 4h,j ; Cell Signalling Technologies 4389, 1:500, Supplementary Fig. 4e ), anti-COX2 (Cell Signalling Technologies, 12282; 1:1,000), anti-phospho ERK (Cell Signalling Technologies, 4377; 1:1,000), anti-total ERK (Cell Signalling Technologies, 9102; 1:1,000) and anti-HNRNP (Santa Cruz Biotechnology, sc-15386; 1:250) and anti-H2 (Cell Signalling, 2595; 1:2,000). Horseradish peroxidase-conjugated anti-mouse and anti-rabbit secondary antibodies were used (Jackson ImmunoResearch Laboratories; 1 h, room temperature). The visualization of immunoreactive proteins was performed with the SuperSignal West Pico Chemiluminescent system (Pierce, 34080), according to the manufacturer’s instructions. Uncropped scans of the immunoblots are included in Supplementary Figs 6 and 7 . The predicted size of GALR2, which does not include post-translational modifications such as glycosylation, is ∼ 42 kDa but we obtain a signal at ∼ 70 kDa. In general, G-protein-coupled receptors, such as GALR2, are heavily glycosylated and multiple bands may be obtained on electrophoresis [63] . The immunoblot with GAL antibody shows a ∼ 13-kDa signal of GAL pre-propeptide, given that the predicted molecular mass of GAL is ∼ 3.1 kDa ( http://www.uniprot.org/uniprot/P22466 ). Invasion assay Cell invasion was quantified 24–48 h after siRNA transfection using Transwell inserts (Corning, 3422) coated with Matrigel (BD Biosciences, 354230), in the modified Boyden chamber chemoinvasion assay. Inserts that were not coated with Matrigel were used as a migration control, and invasion was normalized to migration according to the manufacturer’s instructions by dividing the total number of cells that invaded through Matrigel by the total number of cells that invaded through the control insert. GAL (5 nM, Sigma-Aldrich, G8041) or CM collected from rat DRG cultured in control medium for 48 h was used as a chemoattractant in the lower chamber. Immunohistochemistry and immunofluorescence Human and mouse tumours were stained with anti-COX2 rabbit monoclonal antibody (Cell Signalling Technology, 12282), anti-S100 rabbit polyclonal antibody (Dako, Z0311, used to identify nerves on paraffin-embedded tissue) and cytokeratin AE1/AE3 mouse monoclonal antibody (Pan cytokeratins, EMD Millipore, IHCR2025-6, used to identify tumour cells on paraffin-embedded tissue). Mouse IgG (Dako, X0931) or rabbit IgG (Dako, X0936) was used at the same concentrations as the primary antibodies as a negative control. Biotinylated goat anti-mouse or anti-rabbit secondary antibodies were used (Biocare Medical, GM601 and GR608). Haemotoxylin and eosin staining was performed to assess tumour morphology. Immunofluorescence on frozen CAM sections was performed using human collagen IV antibody [64] (1:1,000) followed by incubation with 4′,6-diamidino-2-phenylindole. Immunofluorescence labelling of neurites was performed as follows: nerve explants were blocked with goat serum and incubated with anti-neurofilament (NF-M 160 kDa chain primary antibody; Zymed Laboratories, 13-0700; 1:500) in 0.3% Triton-X-100, followed by incubation with fluorescent anti-mouse secondary antibody (Jackson ImmunoResearch, 115-006-075). Imaging of representative fields was performed using an Olympus BX-51 microscope. Inclusion and exclusion criteria In most in vivo and in vitro experiments, a normal distribution (in both control and experimental groups) of samples was obtained. However, significant outliers were excluded from analyses. All exclusions were made per predetermined protocol. In vivo models The University of Michigan University Committee on Use and Care of Animals (UCUCA) approved all animal experiments. Mouse Paraffin-embedded tissues from a previously performed animal experiment were used in these studies. As described [7] , 1 × 10 5 OSCC3 cells stably overexpressing GALR2 or control vector (pcDNA) were suspended in Matrigel and injected on the backs of 4–6 week-old athymic mice (Male, Ncr nu/nu strain, NCI, Frederick, n =5), so each mouse had an injection of control and GALR2-overexpressing tumour cells. Animals were euthanized after 14 days. Out of the five animals injected, three palpable tumours were obtained from each group, so subsequent analyses were performed with n =3 per group of control and GALR2-overexpressing tumours. Each tumour generated was used for immunohistochemistry, PNI analysis and nerve quantification. Because previously collected samples were used, no power calculation was performed before analysis. The criteria used for PNI were tumour that approximates the nerve, covering at least 33% of its circumference, or in one of the three layers of the nerve sheath [1] . Chorioallantoic membrane Twenty-four fertilized Lohmann White Leghorn eggs were obtained from the Michigan State University Department of Animal Sciences Poultry Farm for each experiment. The eggs were incubated as described [10] and randomly distributed into treatment groups of six to eight eggs each, and tumour cells were seeded as described [10] . Chicken embryos that did not develop correctly or that were contaminated were excluded from analysis; additionally, control and experimental group tumours outside a normal distribution (significant outliers), were excluded. Exclusions were made per predetermined protocol. In vivo perineural invasion assay DRG were dissected from rats within 1 h of euthanasia and labelled using CellTracker Red CMTPX (Invitrogen, C34552). DRG were seeded on the CAM (day 8) with HNSCC cells (day 10) that were fluorescently labelled with the lipophilic tracer DiO (a dialkylcarbocyanine derivative, 5 μg ml −1 , overnight) before experiments. The CAM was harvested after 48 h (day 12). The neurites were stained using a proprietary stain in the AXIS kit (EMD Millipore, AX15010) according to the manufacturer’s instructions. Tumour spread and neurite outgrowth were imaged using a Leica Stereo microscope and quantified using ImageJ. Neurite outgrowth quantification assay The Neurite Outgrowth Assay Plus kit (EMD Millipore, NS220) was used according to the manufacturer’s instructions. SH-SY5Y human neuroblastoma cells were cultured in DMEM (Gibco, 11965-092) overnight and then 1 × 10 4 cells were seeded on the top chamber of the assay and allowed to project neurites for 48 h. CM from HNSCC cells with or without GAL depletion was used in the lower chamber. Neurites were imaged at 10 × and stained using a proprietary stain from the AXIS kit (EMD Millipore, AX15010) according to the manufacturer’s instructions, and retained dye was solubilized and quantified using a SpectraMax M2e microplate reader and Softmax Pro v5 Software (Molecular Devices). Oncomine analyses The Oncomine database (Life Technologies) was used to collect clinical data used in meta-analyses. A list of neuropeptides ( Table 1 ) based on extensive signalling roles within and outside the neuronal systems [4] , [65] , was generated for comparison across 16 HNSCC studies ( Supplementary Table 1 ). Because PNI status is not included in the information available on Oncomine, survival was used as a surrogate indicator of potential PNI status since poor survival is frequently correlated with PNI [1] , [66] . Each neuropeptide was evaluated for expression in cancer versus normal (non-cancer) tissue and also for 3-year survival versus 3-year death. The studies were dichotomized and studies significant at the 5% level were assigned a value of 1, while insignificant studies were assigned a value of 0. The set was then subjected to a one-sample t -test against a 0.05 expected value. A similar meta-analysis was completed for COX2 expression in cancer versus normal (non-cancer) across 16 HNSCC studies. Studies and corresponding references are listed in Supplementary Table 2 . Proliferation assay Human HNSCC cells (1 × 10 4 ) were plated in triplicate in a 24-well plate. The total number of live cells was quantified every 24 h using trypan blue (Invitrogen, T10282) and a Countess Cell Counter (Invitrogen, C10227). Randomization An effort was made to randomize samples whenever possible in in vivo and in vitro experiments. Chicken embryos were randomized into treatment and control groups. In addition, rat nerves were randomly selected for explant experiments. Mice were not randomized since each mouse received the same two injections (one of control cells and one with GALR2-overexpressing cells). Sample size calculations For CAM experiments, at least a two-fold difference in tumour size, invasion and metastasis was predicted. Therefore, with an α of 0.05, power at 0.8 and coefficient of variation at 0.5 (low due to very consistent tumour seeding and incubation of all samples), at least three CAMs per group was determined to be the minimal sample size. We used six to eight CAMs per group in each experiment. For in vitro experiments, it was similarly predicted that there would be at least a two-fold difference in parameters studied with low variance, so with the same approach described above, we determined that using three replicates per in vitro experiment was appropriate. In vitro experiments were repeated in triplicate or as indicated in the figure legends. How to cite this article: Scanlon, C. S. et al. Galanin modulates the neural niche to favour perineural invasion in head and neck cancer. Nat. Commun. 6:6885 doi: 10.1038/ncomms7885 (2015).